[Au]/[Ag]-catalysed expedient synthesis of branched heneicosafuranosyl arabinogalactan motif ofMycobacterium tuberculosiscell wall Emergence of multidrug-resistant and extreme-drug-resistant strains of Mycobacterium tuberculosis (MTb) can cause serious socioeconomic burdens. Arabinogalactan present on the cellular envelope of MTb is unique and is required for its survival; access to arabinogalactan is essential for understanding the biosynthetic machinery that assembles it. Isolation from Nature is a herculean task and, as a result, chemical synthesis is the most sought after technique. Here we report a convergent synthesis of branched heneicosafuranosyl arabinogalactan (HAG) of MTb. Key furanosylations are performed using [Au]/[Ag] catalysts. The synthesis of HAG is achieved by the repetitive use of three reactions namely 1,2- trans furanoside synthesis by propargyl 1,2-orthoester donors, unmasking of silyl ether, and conversion of n -pentenyl furanosides into 1,2-orthoesters. Synthesis of HAG is achieved in 47 steps (with an overall yield of 0.09%) of which 21 are installation of furanosidic linkages in a stereoselective manner. M ycobacterium tuberculosis (MTb) is the causative agent of Tuberculosis, the deadly disease that is plaguing mankind [1] , [2] , [3] , [4] , [5] , [6] . Robert Koch noticed that MTb has a thick and waxy cellular envelope, which was later shown to not only act as a large obstruction to the entry of antibiotics but also modulate the host immune system [3] , [4] . Some of the currently administered frontline drugs are demonstrated to inhibit the biosynthesis of cell wall [7] , [8] . The complete structure of the cell wall of MTb has been unravelled to observe that it has two major components termed as mycolylarabinogalactan and lipoarabinomannan wherein arabinose and galactose are in furanosyl and mannose in the pyranosyl form [9] , [10] , [11] , [12] , [13] , [14] . Ara f - and Gal f - are xenobiotic to humans and, therefore, understanding the biosynthesis of the cell wall components containing them is of particular significance for developing novel therapeutic agents [12] . Prospect of biological significance coupled with the challenge of large oligofuranosides synthesis has cajoled many synthetic carbohydrate chemists to develop strategies for assembling AG and lipoarabinomannan fragments [15] , [16] , [17] , [18] , [19] , [20] , [21] , [22] , [23] , [24] , [25] , [26] , [27] , [28] , [29] . Synthesis of oligosaccharides is an art of its own and each synthesis poses a unique challenge and demands deployment of multiple glycosyl donors [30] , [31] , [32] . To date, the largest fragment of the mycobacterial arabinogalactan was synthesized independently by groups headed by Lowary and Ito; but without Gal f residues ( Fig. 1 ) [33] , [34] . 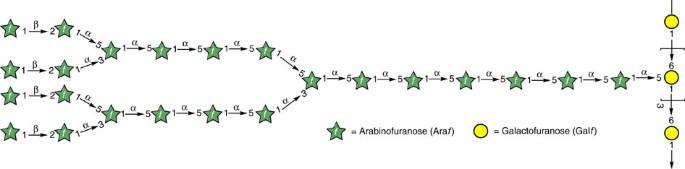Figure 1: Arabinogalactan motif ofMycobacterium tuberculosiscell wall. Arabinan is attached at the C-5 position of the galactan. Both arabinose and galactose are in the furanosyl form. Galf(1→6)Galflinkages and Araf(1→3 or 5)Araflinkages are all in the 1,2-transmanner, whereas Araf(1→2)Araflinkages are1,2-cis mannered. Figure 1: Arabinogalactan motif of Mycobacterium tuberculosis cell wall. Arabinan is attached at the C-5 position of the galactan. Both arabinose and galactose are in the furanosyl form. Gal f (1→6)Gal f linkages and Ara f (1→3 or 5)Ara f linkages are all in the 1,2- trans manner, whereas Ara f (1→2)Ara f linkages are 1 ,2-cis mannered. Full size image In this Article, we show that the highly branched heneicosafuranosyl arabinogalactan (HAG) can be synthesized by the repeated use of gold-catalysed activation of alkynyl 1,2- O -orthoester chemistry that was developed in our laboratory [35] , [36] , [37] , [38] , [39] , [40] . Retrosynthesis Retrosynthetic disconnections of heneicosafuranoside 1 recognized that the assembly of heneicosafuranoside requires four major constituents namely cassettes A–D ( Fig. 2 ). Heneicosafuranoside 1 can be synthesized by the 1,2- trans diastereoselective furanosylation between propargyl 1,2-orthoester of tetrasaccharide 2 and the tridecasaccharide-aglycon under gold-catalysed glycosidation conditions. Synthesis of tridecasaccharide 3 can be envisaged from 1,2-orthoester of a hexasaccharide cassette B ( 4 ) and the heptasaccharide-aglycon 5 . Heptasaccharide synthesis can be realized by the gold-catalysed furanosylation between a tetraarabinofuranosyl orthoester cassette C ( 6 ) and the trisaccharide cassette D ( 7 ). Synthesis of cassettes A–D is envisioned from building blocks 8a – 8d , 9 , 10 . Propargyl 1,2-orthoesters are envisioned from corresponding n -pentenyl glycosides wherein n -pentenyl moiety serves as an excellent protecting group that can be transformed to anomeric bromide in transit to the orthoester preparation [38] , [41] . 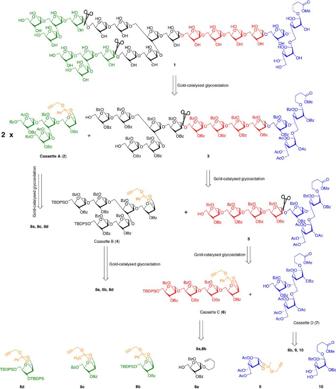Figure 2: Retrosynthetic plan for the synthesis of heneicosafuranoside 1. Retrosynthetic analysis shows the assembly of heneicosafuranosyl arabinogalactan (1) can be synthesized from cassettes A-D which in turn can be obtained from monosaccharides8a–8d,9and10. Figure 2: Retrosynthetic plan for the synthesis of heneicosafuranoside 1. Retrosynthetic analysis shows the assembly of heneicosafuranosyl arabinogalactan ( 1 ) can be synthesized from cassettes A-D which in turn can be obtained from monosaccharides 8a – 8d , 9 and 10 . Full size image Synthesis of monosaccharide-building blocks HAG synthesis started with the development of methods for the large-scale synthesis of building blocks 8a – 8d ( Fig. 3 ). Easily accessible 1,2-orthoester 11 (ref. 36 ) was saponified under Zemplén deacetylation conditions to afford a diol, which was treated with one molar equivalent of TBDPS-Cl to get the alcohol 12 . A portion of the compound 12 was esterified using BzCl/py to obtain building block 8b (see Supplementary Figs 1–3 ) and the remaining portion was converted into disilyl ether 8d (see Supplementary Figs 7–9 ). 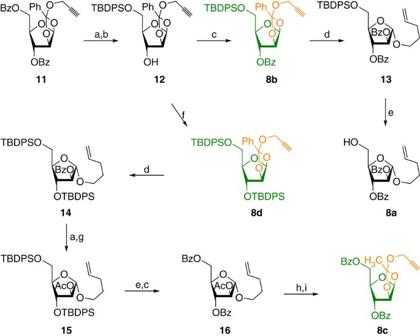Figure 3: Synthesis of arabinofuranoside-building blocks. Reagents and conditions: (a) NaOMe, MeOH, 25 °C, 6 h. (b) TBDPS-Cl (1 eq.), imidazole,N,N′-dimethylformamide (DMF), 0→25 °C, 12 h. (c) BzCl, Et3N, CH2Cl2, 0 °C→25 °C, 61%: three steps for8bfrom11. (d) Pent-4-enol, AuCl3, 4 Å MS, CH2Cl2, 25 °C, 2 h. (e) Py·HF, THF:Py (5:1), 0 °C→25 °C, 5 h, 66%: two steps for8afrom8b. (f) TBDPS-Cl (1 eq.), Imidazole, DMF, 25 °C, 10 h, 74%: two steps for8dfrom11. (g) Ac2O, pyridine, 0 °C→25 °C. (h) Br2, CH2Cl2, 4 Å MS, 0 °C, 15 min. (i) Propargyl alcohol, 2,6-lutidine, CH2Cl2, 4 Å MS, 0 °C →25 °C, 10 h, overall 57% from8d. Figure 3: Synthesis of arabinofuranoside-building blocks. Reagents and conditions: (a) NaOMe, MeOH, 25 °C, 6 h. (b) TBDPS-Cl (1 eq. ), imidazole, N , N ′-dimethylformamide (DMF), 0→25 °C, 12 h. (c) BzCl, Et 3 N, CH 2 Cl 2 , 0 °C→25 °C, 61%: three steps for 8b from 11 . (d) Pent-4-enol, AuCl 3 , 4 Å MS, CH 2 Cl 2 , 25 °C, 2 h. (e) Py·HF, THF:Py (5:1), 0 °C→25 °C, 5 h, 66%: two steps for 8a from 8b . (f) TBDPS-Cl (1 eq. ), Imidazole, DMF, 25 °C, 10 h, 74%: two steps for 8d from 11 . (g) Ac 2 O, pyridine, 0 °C→25 °C. (h) Br 2 , CH 2 Cl 2 , 4 Å MS, 0 °C, 15 min. (i) Propargyl alcohol, 2,6-lutidine, CH 2 Cl 2 , 4 Å MS, 0 °C →25 °C, 10 h, overall 57% from 8d . Full size image Further, gold-catalysed glycosidation conditions [36] were employed on glycosyl donor 8b to obtain n -pentenyl furanoside 13 followed by the deprotection of TBDPS group using Py·HF to obtain the desired building block 8a in very high yields. Gold-catalysed glycosidation between orthoester 8d and 4-penten-1-ol resulted into the n -pentenyl furanoside 14 , which was subsequently transformed into acetate 15 . Deprotection of silyl ethers in presence of Py·HF followed by esterification afforded the compound 16 . n -Pentenyl furanoside 16 was converted into the 1,2-orthoester-building block 8c employing a recently established protocol [38] . Compound 16 was treated with Br 2 /CH 2 Cl 2 /4 Å mass spectrometry (MS) at 0 °C for 15 min to obtain the glycosyl bromide that was immediately treated with propargyl alcohol and 2,6-lutidine to afford the building block 8c in 85% yield over two steps (see Supplementary Figs 4–6 ). Galactofuranoside 17 (ref. 42 ) was uneventfully converted into orthoester 9 in two steps followed by the gold-catalysed furanosylation to afford compound 18 that was converted into building block 10 in four steps namely saponification of compound 18 resulting into a tetraol, locking of C -5 and C -6 hydroxyls as isopropylidene using 2-methoxypropene/ p -Toluenesulfonic acid (PTSA) in dichloromethane, esterification of C -2 and C -3 hydroxyl groups, and cleavage of isopropylidene using PTSA in MeOH with an overall yield of 70% (see Supplementary Figs 13–15 ; Fig. 4 ). Conversion of n -pentenyl furanosides into propargyl 1,2-orthoesters is considered to increase the reactivity of the donor and also conduct the reactions under catalytic conditions [38] . 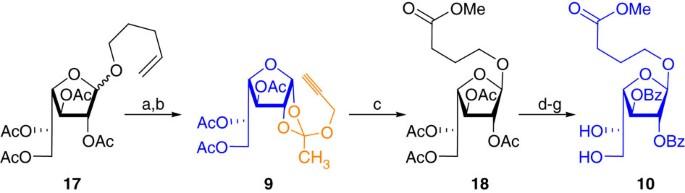Figure 4: Synthesis of Galactofuranoside-building blocks. Reagents and conditions: (a) Br2, CH2Cl2, 4 Å MS, 0 °C, 15 min. (b) Propargyl alcohol, 2,6-lutidine CH2Cl2, 4 Å MS 0 °C→25 °C, 10 h, 81% over two steps. (c) Methyl 4-hydroxybutanoate, AuCl3, 4 Å MS, CH2Cl2, 25 °C, 2 h, 80%. (d) NaOMe, MeOH, 25 °C, 15 h. (e) 2-Methoxypropene, acetone, PTSA, 8 h. (f) BzCl, py., 0→25 °C. (g) PTSA, MeOH, 25 °C, 4 h, 70% over four steps. Figure 4: Synthesis of Galactofuranoside-building blocks. Reagents and conditions: (a) Br 2 , CH 2 Cl 2 , 4 Å MS, 0 °C, 15 min. (b) Propargyl alcohol, 2,6-lutidine CH 2 Cl 2 , 4 Å MS 0 °C→25 °C, 10 h, 81% over two steps. (c) Methyl 4-hydroxybutanoate, AuCl 3 , 4 Å MS, CH 2 Cl 2 , 25 °C, 2 h, 80%. (d) NaOMe, MeOH, 25 °C, 15 h. (e) 2-Methoxypropene, acetone, PTSA, 8 h. (f) BzCl, py., 0→25 °C. (g) PTSA, MeOH, 25 °C, 4 h, 70% over four steps. Full size image Synthesis of cassettes A–D Synthesis of Heneicosafuranoside commenced with the preparation of cassettes A–D. Towards this affect, one molar equivalent of Gal f orthoester 9 was added dropwise to a solution of diol 10 in CH 2 Cl 2 and allowed to react under standard gold-catalysed glycosidation conditions to obtain the Gal f (1→6)β-Gal f disaccharide regioselectively in 70% yield. In continuation, the first arabinofuranosyl residue was attached at the C -5 hydroxyl group of disaccharide 19 under gold-catalysed conditions using the orthoester 8b to afford the arabinogalactan 20 in 85% yield, which was converted to cassette D ( 7 ) by F-mediated cleavage of silyl ether ( Fig. 5 ). 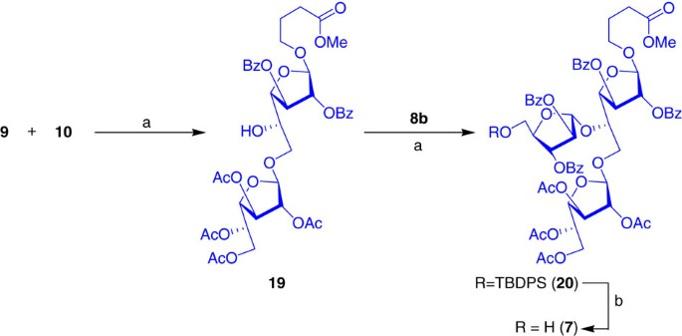Figure 5: Synthesis of cassette D. Reagents and conditions: (a) AuCl3(7 mol%), AgOTf (7 mol%), CH2Cl2, 4 Å MS powder, 25 °C, 2 h; 70% for19and 75% for20. (b) Py·HF, THF:Py (5:1), 0 °C→25 °C, 4 h, 95%. Figure 5: Synthesis of cassette D. Reagents and conditions: (a) AuCl 3 (7 mol%), AgOTf (7 mol%), CH 2 Cl 2 , 4 Å MS powder, 25 °C, 2 h; 70% for 19 and 75% for 20 . (b) Py·HF, THF:Py (5:1), 0 °C→25 °C, 4 h, 95%. Full size image Synthesis of cassette C ( 6 ) commenced with the gold-catalysed glycosidation reaction between donor 8a and aglycon 8b in CH 2 Cl 2 to obtain disaccharide 21 (ref. 38 ). Deprotection of silyl ether resulted in the aglycon 22 and the treatment of disaccharide 21 with Br 2 in CH 2 Cl 2 followed by propargyl alcohol and 2,6-lutidine, TBAI afforded the glycosyl donor 23 in 85% yield. An uneventful reaction between aglycon 22 and donor 23 employing AuCl 3 /AgOTf conditions afforded the tetrasaccharide 24 , which was converted into cassette C ( 6 ) in two well-optimized steps ( Fig. 6 ). 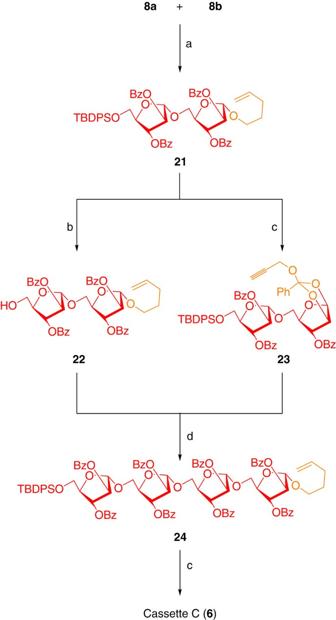Figure 6: Synthesis of cassette C. Reagents and conditions: (a) AuCl3(7 mol%), CH2Cl2, 4 Å MS powder, 25 °C, 2 h, 84%. (b) Py·HF, THF:Py (5:1), 0 °C→25 °C, 4 h, 95%. (c) Br2, CH2Cl2, 4 Å MS powder, 10 min, 0 °C followed by propargyl alcohol, 2,6-lutidine, tetrabutylammonium iodide, 0 °C→25 °C, 12 h, 85% for23and 88% for6. (d) AuCl3(7 mol%), AgOTf (7 mol%), CH2Cl2, 4 Å MS powder, 25 °C, 12 h, 84%. Figure 6: Synthesis of cassette C. Reagents and conditions: (a) AuCl 3 (7 mol%), CH 2 Cl 2 , 4 Å MS powder, 25 °C, 2 h, 84%. (b) Py·HF, THF:Py (5:1), 0 °C→25 °C, 4 h, 95%. (c) Br 2 , CH 2 Cl 2 , 4 Å MS powder, 10 min, 0 °C followed by propargyl alcohol, 2,6-lutidine, tetrabutylammonium iodide, 0 °C→25 °C, 12 h, 85% for 23 and 88% for 6 . (d) AuCl 3 (7 mol%), AgOTf (7 mol%), CH 2 Cl 2 , 4 Å MS powder, 25 °C, 12 h, 84%. Full size image En voyage to the synthesis of heneicosafuranoside 1 , synthesis of cassettes A and B continued with the successful synthesis of disaccharide 25 from arabinofuranosyl donor 8d and aglycon 8a . n -Pentenyl disaccharide 25 was converted to diol 26 under Py·HF/THF/4 h/80% and reacted with donor 8b (2.5 eq.) to obtain a tetrasaccharide 27 , which was converted into a diol that was immediately treated with 2.5 molar equivalents of donor 8b to afford the hexasaccharide 28 commissioning gold-catalysed glycosidation conditions. Finally, conversion of n -pentenyl furanoside was converted into the cassette B ( 4 ) in two steps by reacting with Br 2 /CH 2 Cl 2 /4 Å MS/0 °C/15 min followed by propargyl alcohol/2,6-lutidine/CH 2 Cl 2 /4 Å MS/0→25 °C/10 h in 86% yield over two steps. Similarly, diol 26 was treated with donor 8c (2.5 eq.) to obtain a tetrasaccharide 29 , which was converted into cassette A ( 2 ) via glycosyl bromide intermediate ( Fig. 7 ). 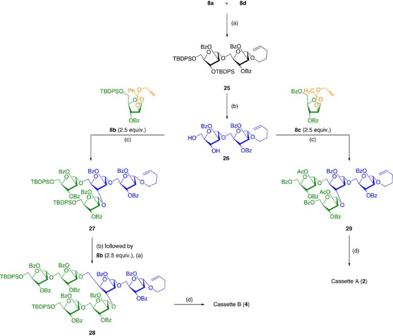Figure 7: Synthesis of cassettes A and B. Reagents and conditions: (a) AuCl3(7 mol%), CH2Cl2, 4 Å MS powder, 25 °C, 2 h, 81% for25and 50% for28. (b) Py·HF, THF:Py (5:1), 0 °C→25 °C, 4 h, 80% for26and 75% for28. (c) AuCl3(7 mol%), AgOTf (7 mol%), CH2Cl2, 4 Å MS powder, 25 °C, 2 h, 48% for29and 45% for27. (d) Br2, CH2Cl2, 4 Å MS powder, 10 min, 0 °C followed by propargyl alcohol, 2,6-lutidine, tetrabutylammonium iodide, 0 °C→25 °C, 12 h, 88% for2and 86% for4. Figure 7: Synthesis of cassettes A and B. Reagents and conditions: (a) AuCl 3 (7 mol%), CH 2 Cl 2 , 4 Å MS powder, 25 °C, 2 h, 81% for 25 and 50% for 28 . (b) Py·HF, THF:Py (5:1), 0 °C→25 °C, 4 h, 80% for 26 and 75% for 28 . (c) AuCl 3 (7 mol%), AgOTf (7 mol%), CH 2 Cl 2 , 4 Å MS powder, 25 °C, 2 h, 48% for 29 and 45% for 27 . (d) Br 2 , CH 2 Cl 2 , 4 Å MS powder, 10 min, 0 °C followed by propargyl alcohol, 2,6-lutidine, tetrabutylammonium iodide, 0 °C→25 °C, 12 h, 88% for 2 and 86% for 4 . Full size image Synthesis of HAG In continuation of this expedition, gold-catalysed glycosidation between donor cassette C ( 6 ) and acceptor cassette D ( 7 ) afforded the heptasaccharide ( 30 ) containing five Ara f - residues and two Gal f - residues in 1,2- trans disposition. The successful synthesis of heptasaccharide was confirmed by the 13 C NMR spectral studies, wherein all seven anomeric carbons of compound 30 were noticed between 105.3 and 106.7 p.p.m. (see Supplementary Fig. 59 ). The C -5 hydroxyl group at the non-reducing end of heptasaccharide 30 was unmasked by the addition of Py·HF in THF to obtain alcohol 5 , which was coupled with n -pentenyl donor 28 to obtain the required tridesaccharide 31 in 24% yield after 4 days. However, the reaction between heptasaccharide 5 and cassette B ( 4 ) under the standard gold-catalysed conditions afforded tridecaoligosaccharide 31 in 65% yield ( Fig. 8 ). 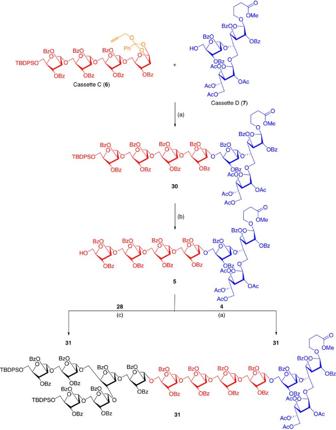Figure 8: Synthesis of tridecaoligofuranoside. Reagents and conditions: (a) AuCl3(7 mol%), AgOTf (7 mol%), CH2Cl2, 4 Å MS powder, 25 °C, 24 h, 70% for30and 65% for31. (b) Py·HF, THF:Py (5:1), 0 °C→25 °C, 4 h, 85% (c) NIS (3 eq.), TfOH (0.3 eq.), 4 days, 0 °C→25 °C, 24%. Figure 8: Synthesis of tridecaoligofuranoside. Reagents and conditions: (a) AuCl 3 (7 mol%), AgOTf (7 mol%), CH 2 Cl 2 , 4 Å MS powder, 25 °C, 24 h, 70% for 30 and 65% for 31 . (b) Py·HF, THF:Py (5:1), 0 °C→25 °C, 4 h, 85% (c) NIS (3 eq. ), TfOH (0.3 eq. ), 4 days, 0 °C→25 °C, 24%. Full size image Unmasking of the silyl ether using Py·HF/THF afforded the glycosyl acceptor 3 that can be glycosylated with a tetrasaccharide-donor cassette A ( 2 ). The gold-catalysed glycosidation between acceptor 3 and 2.5 equivalents of the donor 2 was performed at 25 °C for 24 h to afford the HAG ( 32 ) in fully protected form. In the 1 H NMR spectrum, all singlets between δ 4.97–5.75 p.p.m. indicated the presence of all 1,2- trans linkages at the anomeric position and in the 13 C NMR spectrum, resonances due to 21-anomeric carbons appeared between δ 105.2–106.7 p.p.m. (see Supplementary Fig. 71 ). Further, matrix-assisted laser desorption/ionization–time of flight–mass spectrometry (MALDI–TOF–MS) also supported the formation of HAG ( 32 ) of MTb cell surface ( Fig. 9 ). Zemplèn deacylation using 0.5 M NaOMe in MeOH afforded the fully deprotected HAG with methyl butanoate linker at the reducing end. In the 1 H and 13 C NMR spectra, resonances due to the benzoate moiety completely disappeared. The 150 MHz 13 C NMR spectrum showed signals at δ 176.9, 52.2, 30.6 (−CH 2 ), 24.2 (−CH 2 ) p.p.m. confirmed the presence of the methyl butanoate linker at the reducing end. Resonances in the anomeric region did not resolve fully for complete assignment even at this field, although two resonances at δ 108.60 and 108.63 p.p.m. confirmed the presence of two β-Gal f - residues on the basis of previous assignments (see Supplementary Figs 72,73 ). In addition, the high-resolution MALDI–TOF mass spectrum of compound 1 showed a molecular ion of the sodium adduct at m/z =2,974.2810 (see Supplementary Fig. 74 ), matching satisfactorily with that of calculated exact mass of compound 1 . 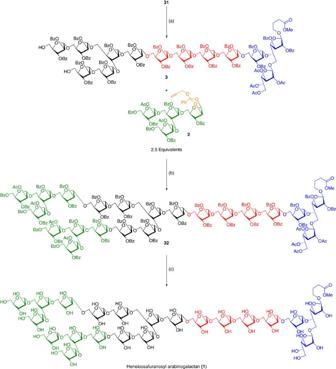Figure 9: Synthesis of heneicosafuranosyl arabinogalactan (1). Reagents and conditions: (a) Py·HF, THF:Py (5:1), 0 °C→25 °C, 4 h, 85%. (b) AuCl3(7 mol%), AgOTf (7 mol%), CH2Cl2, 4 Å MS powder, 25 °C, 24 h, 71%. (c) 0.5M NaOMe, MeOH, CH2Cl2, 4 h, 25 °C, 74%. Figure 9: Synthesis of heneicosafuranosyl arabinogalactan (1). Reagents and conditions: (a) Py·HF, THF:Py (5:1), 0 °C→25 °C, 4 h, 85%. (b) AuCl 3 (7 mol%), AgOTf (7 mol%), CH 2 Cl 2 , 4 Å MS powder, 25 °C, 24 h, 71%. (c) 0.5M NaOMe, MeOH, CH 2 Cl 2 , 4 h, 25 °C, 74%. Full size image In summary, the synthesis of HAG containing nineteen 1,2- trans -Ara f s and two Gal f s was successfully achieved by utilizing Au/Ag-catalysed furanosylations in 0.09% overall yield. The key features associated with this effort are: (1) the stereoselective installation of 1,2- trans Ara f - and Gal f - residues using propargyl 1,2-orthoesters as glycosyl donors, (2) all glycosylation reactions were catalytic, high yielding and thus easy to purify, (3) the convergent fragment coupling between linear/branched oligosaccharides using propargyl 1,2- O -orthoester donor chemistry. Essentially, the expedient synthesis of HAG built on only three repetitive reactions namely glycosidation in the presence of catalytic amount of AuCl 3 and AgOTf; cleavage of O -silyl ether using Py·HF; and transformation of n -pentenyl glycosides into 1,2-orthoesters. The whole synthesis is modular and thus amenable for the synthesis of various saccharide mutants for eliciting the biological response. General methods Unless otherwise noted, materials were obtained from commercial suppliers and were used without further purification. Unless otherwise reported, all reactions were performed under Argon atmosphere. Removal of solvent in vacuo refers to distillation using a rotary evaporator attached to an efficient vacuum pump. Products obtained as solids or syrups were dried under a high vacuum. Gold and silver salts were purchased from Sigma-Aldrich India Limited. Amberlite was purchased from Sigma-Aldrich and Bio-gel P-4 gel was purchased from Bio-Rad Laboratories, USA. Analytical thin-layer chromatography was performed on pre-coated silica plates (F 254 , 0.25 mm thickness) from Merck; compounds were visualized by ultraviolet light or by staining with anisaldehyde spray. Optical rotations were measured on a JASCO 2000 P digital polarimeter. Infrared spectra were recorded on a Bruker Fourier transform infrared spectrometer. NMR spectra were recorded either on a Bruker Avance 400 or a 500 or 600 MHz with CDCl 3 or D 2 O as the solvent and tetramethylsilane as the internal standard. High-resolution mass spectroscopy was performed using ABI MALDI–TOF or Waters Synapt G2 ESI mass analyser. Low-resolution mass spectroscopy was performed on Waters ultra performance liquid chromatography (UPLC)-MS, and thin-layer chromatography MS was checked on SWADESI-TLC MS interface. A small quantity (5–10%) of propargyl glycosides was observed in most of the gold-catalysed glycosidations with propargyl orthoesters as reported earlier [35] . For NMR analysis and high-resolution mass spectrometry of the compounds in this article, see Supplementary Figs 1–74 . Gold(III)-catalysed 1,2- trans glycosidation To a CH 2 Cl 2 solution (5 ml) containing glycosyl donor (0.1–1 mmol) and aglycon (0.1–1 mmol)) with 4 Å molecular sieves powder (0.1–1.0 g) was added a catalytic amount of AuCl 3 (7 mol%; AgOTf (7 mol%) as an additive wherever mentioned) and stirred at 25 °C (ref. 37 ). After 2 h (for oligosaccharides up to 24 h), the reaction mixture was neutralized by the addition of Et 3 N and filtered through a pad of celite and concentrated in vacuo . The resulting residue was purified by silica gel column chromatography using ethyl acetate-petroleum ether to obtain 1,2- trans glycosides as a fluffy solids. Glycosidation by n -pentenyl glycosides To a CH 2 Cl 2 solution (5 ml) containing glycosyl donor (0.1–1 mmol) and aglycon (0.1–1 mmol)) with 4 Å molecular sieves powder (0.1–1.0 g) was added 3 molar eq. of N -iodosuccinimide (NIS) at 0 °C in ice bath and stirred for 10 min [21] . After 10 min, catalytic amount of TfOH (0.3 eq.) was added to the reaction mixture at 0 °C and stirred at 25 °C. After complete disappearance of the donor (adjudged by TLC), the reaction mixture was neutralized by the addition of Et 3 N and filtered through a pad of celite. The filtrate was washed with sat. aqueous solutions of sodium bicarbonate and sodium thiosulphate. Combined organic layers were dried over sodium sulphate and concentrated in vacuo . The resulting residue was purified by flash silica gel column chromatography using ethyl acetate-petroleum ether to obtain 1,2- trans glycosides. Pent-4-enyl glycosides to propargyl orthoesters Pent-4-enyl furanoside (1–50 mmol) was dissolved in anhydrous CH 2 Cl 2 (10–500 ml) and cooled to 0 °C (ref. 38 ). Br 2 (1.1 molar eq.) in CH 2 Cl 2 was added dropwise to the reaction mixture with constant stirring at 0 °C. In addition, the reaction mixture was stirred for 10 min at 0 °C and concentrated under reduced pressure to give furanosyl bromide as white foam, which was immediately used in the next step without further purification. The crude furanosyl bromide was redissolved (10–500 ml) in anhydrous CH 2 Cl 2 , propargyl alcohol (1.5–2 molar eq.) and 2,6-lutidine (2–3 molar eq). Catalytic amount of tetra n -butyl ammonium iodide was added to the reaction and stirred for 4 h to overnight at room temperature. The reaction mixture was diluted with CH 2 Cl 2 (100–500 ml) and water (100–500 ml), and the aqueous layer was extracted with CH 2 Cl 2 (2 x ), the organic extract was washed with saturated oxalic acid solution and saturated sodium bicarbonate solution. The organic phase was collected, dried over sodium sulphate and concentrated in vacuo . Crude residue of the orthoester was purified by silica gel column chromatography (EtOAc:petroleum ether) to obtain propargyl 1,2- O -orthoester as a white foam/solid. Cleavage of O -silyl ethers To a solution of O -TBDPS protected saccharide (0.1–10 mmol) in THF:py (10:2–100:20 ml) was added Py·HF (2 molar eq. per O -TBDPS) and the reaction mixture was stirred at 25 °C for 4–12 h (ref. 38 ). The reaction was arrested by adding saturated aqueous solution of NaHCO 3 and extracted with EtOAc. The EtOAc layer was dried over anhydrous sodium sulphate and concentrated in vacuo . The crude residue was purified by flash column chromatography (EtOAc:petroleum ether) using silica gel. Deprotection of benzoates A 0.5 M NaOMe in MeOH (2 ml) was added to a solution of compound 32 (110 mg, 15.4 μmol) in 1:1 MeOH-CH 2 Cl 2 (4 ml) and stirred at 25 °C. After 4 h, the reaction mixture was quenched by the addition of Amberlite-IR120 (H + ) resin, filtered and the filtrate was concentrated in vacuo to obtain a residue that was washed sequentially with chloroform and ethyl acetate to remove majority of the methyl benzoate. The remaining residue was purified by column chromatography using Bio-gel-P4 gel (90–180 μm, exclusion limit 4,000 Da). The compound was collected using Millipore water, concentrated in vacuo and further lyophilized for 24 h to obtain the HAG 1 (34 mg, 74%) as a white solid. Data availability The authors declare that some of the data supporting the findings of this study are available in its Supplementary Information files. All data are available from the authors upon reasonable request. How to cite this article: Thadke, S. A. et al . [Au]/[Ag]-catalysed expedient synthesis of branched heneicosafuranosyl arabinogalactan motif of Mycobacterium tuberculosis cell wall. Nat. Commun. 8, 14019 doi: 10.1038/ncomms14019 (2017). Publisher’s note: Springer Nature remains neutral with regard to jurisdictional claims in published maps and institutional affiliations.